Habitat changes and changing predatory habits in North American fossil canids The spread of open grassy habitats and the evolution of long-legged herbivorous mammals with high-crowned cheek teeth have been viewed as an example of coevolution. Previous studies indicate that specialized predatory techniques in carnivores do not correlate with the spread of open habitats in North America. Here we analyse new data on elbow-joint shape for North American canids over the past ∼ 37 million years and show that incipiently specialized species first appeared along with the initial spread of open habitats in the late Oligocene. Elbow-joint morphologies indicative of the behavior of modern pounce-pursuit predators emerged by the late Miocene coincident with a shift in plant communities from C 3 to C 4 grasses. Finally, pursuit canids first emerged during the Pleistocene. Our results indicate that climate change and its impact on vegetation and habitat structure can be critical for the emergence of ecological innovations and can alter the direction of lineage evolution. The future effect of anthropogenic climate change on current biodiversity is a matter of significant concern [1] , [2] , [3] . However, although predictive models can give important clues to short-term biotic reactions [4] , [5] , only the fossil record can provide empirical data on evolutionary responses during long periods of profound climatic and environmental change [6] , [7] , [8] , [9] . Here we demonstrate that the evolution of predatory behaviour in North American canids (for example, foxes and wolves; family Canidae) has been influenced by climatic and environmental transformation over the later Cenozoic (the past ∼ 37 million years (Myr ago)). During this time, Earth’s climate underwent a profound transition in higher latitudes, from climates that were warmer and more humid than today to a later cooling which resulted in increasingly modern climatic regimes [10] . This climatic trend was also accompanied by a marked transition in vegetation structure indicative of increasingly open habitats over the more forested ones [11] . Plant silica microfossils (phytoliths) attest that open-habitat grasslands were well established in North America by the end of the Oligocene at ∼ 27–23 Myr ago [12] . This trend towards habitat opening had a strong impact on mammalian palaeocommunities, as evidenced by changes in ungulate (hoofed mammals) craniodental morphology indicative of feeding on more abrasive forage (for example, hypsodont (high-crowned) cheek teeth), and changes in limb morphology to the elongate limbs typical of present-day fast-running (cursorial) open-habitat ungulates [8] , [13] , [14] . However, while large herbivores are the faunal components directly impacted by vegetational change, the effect of such changes on large carnivores has been less studied. Some previous studies suggest that carnivores with limb morphology indicative of fast running did not evolve until the Pliocene [13] , [15] , [16] , and therefore ∼ 20 Myr ago after the initial spread of open grassy habitats and the evolution of the long-legged ungulates. Here we use the impressive and well-documented fossil record of North American canids [17] , [18] , [19] to test if their inferred locomotor/predatory behaviour was influenced by Cenozoic environmental change towards open habitats, as has been documented in the contemporaneous large herbivores [8] , [11] , [14] . We test for direct association between predatory behaviour and environmental events, rather than an ‘arms-race’ hypothesis between predators and prey. We use statistical shape analysis on two-dimensional (2D) anatomical landmarks drawn from the anterior surface of the humeral distal epiphysis to analyse the shape of the elbow-joint in extinct canids ( Fig. 1a ), ranging from the Oligocene ( ∼ 37 Myr ago) to the end of the Pleistocene ( ∼ 0.01 Myr ago), in comparison with a large sample of modern carnivores of known predatory behaviour. We analyse the shape of the elbow-joint because it is an established morphological indicator of locomotor/predatory behaviour in living carnivores [20] , [21] , [22] , as it reflects the relative range of forearm motion ( Fig. 1b ). Whereas ambush predators need to retain supinatory ability (that is, rotation of the manus to palm-upwards position) to grapple with prey, both pursuit (long-distance running [23] ) and pounce-pursuit (short-distance sprinting [23] ) carnivores have forelimbs with the manus more locked into a prone position, and limb movement more restricted to the parasagittal plane [21] , [22] . 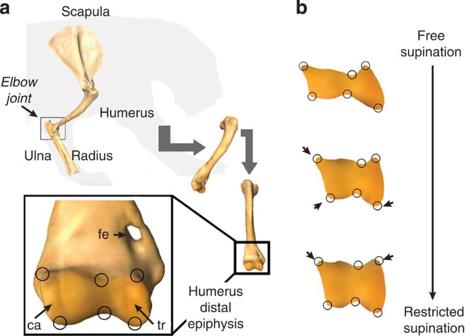Figure 1: The elbow-joint structure. (a) Anatomy of the elbow-joint exemplified in a 3D model ofPanthera onca(jaguar) showing the six 2D-landmarks digitized (circles) to capture the shape of the anterior surface of the humerus distal epiphysis (elbow joint) of living predators and extinct canids. (b) Elbow-joint shape differences between the three present-day predatory groups. From up to down:Panthera tigris(ambush predator),Vulpes vulpes(pounce-pursuit predators) and,Lycaon pictus(pursuit predator). fe, entepicondylar foramen; ca, capitulum; tr, trochlea. Figure 1: The elbow-joint structure. ( a ) Anatomy of the elbow-joint exemplified in a 3D model of Panthera onca (jaguar) showing the six 2D-landmarks digitized (circles) to capture the shape of the anterior surface of the humerus distal epiphysis (elbow joint) of living predators and extinct canids. ( b ) Elbow-joint shape differences between the three present-day predatory groups. From up to down: Panthera tigris (ambush predator), Vulpes vulpes (pounce-pursuit predators) and, Lycaon pictus (pursuit predator). fe, entepicondylar foramen; ca, capitulum; tr, trochlea. Full size image The study confirms that the elbow joints of canids became increasingly modified towards morphology indicative of fast-running predatory behaviour in correlation with the progressive spread of grasslands in the later Cenozoic. We specifically show that: (i) early Oligocene canids were all generalized ambushers; (ii) more cursorial borophagine canids incipiently specialized towards pounce-pursuit predation appeared along with the initial spread of open habitats in the late Oligocene; (iii) although a second incipient specialization towards pounce-pursuit predation appeared within early cursorial canine canids, morphologies of modern specialized pounce-pursuit predators appeared in the late Miocene ( ∼ 7 Myr ago), coincident with a shift in plant communities from C 3 to C 4 grasses [24] ; and (iv) true pursuit and endurance canids only appeared with the colder and more arid conditions of the Pleistocene ( ∼ 2 Myr ago). Our results demonstrate that climate change and its impact on vegetation and habitat structure can be critical for the emergence of ecological innovations and can alter the direction of lineage evolution. Assessing the phylogenetic signal in elbow size and shape The permutation test performed to assess for the presence of phylogenetic structure in the elbow-joint ( Fig. 1 ), using the phylogeny shown in Supplementary Fig. 1 gave statistically significant results for both elbow size (Permutation test for phylogenectic signal; Tree length: 3.766; P -value: <0.0001; 10,000 rounds) and shape (Permutation test for phylogenetic signal; Tree length: 0.226; P -value: <0.0001; 10,000 rounds). Furthermore, the multivariate regression of elbow shape on size was highly significant (Permutation test; N =59; P -value: 0.0002; 10,000 rounds) with a percentage of elbow shape explained for by size differences of 15.09%, which indicates an effect of interspecific allometry. However, the multivariate regression of both contrasted variables after accounting for phylogenetic effects was not significant (Permutation test; N =58; P -value: 0.7564; 10,000 rounds), indicating an absence of evolutionary allometry. Furthermore, the phylogenetic signal of the size-free shape residuals was also significant (Permutation test for phylogenetic signal; Tree length=0.2339; P <0.0001; 10,000 rounds). Therefore, the significant correlation of shape on size obtained above was due to phylogenetic patterning, and thus size-correction of the data was not necessary. For this reason, we employed the Procrustes coordinates (Proc) of elbow shape in subsequent multivariate analyses. The regressions performed between the independent contrasts and their s.d. yielded a non-significant result for both elbow shape (Permutation test; N =58; P -value=0. 6804; 10,000 rounds) and centroid size (Permutation test; N =58; P -value=0.8721; 10,000 rounds), which indicates that our shape and size data and our assembled tree fit adequately [25] and demonstrates that the independent contrast analyses were correctly made. Predatory behaviour The canonical variate analysis (CVA) performed from the Procrustes coordinates (Proc) of elbow shape using the extant sample ( Table 1 ) yielded two canonical functions (canonical axis I: λ =3.01, variance (%)=83.4; canonical axis II: λ =0.659, variance (%)=16.6). 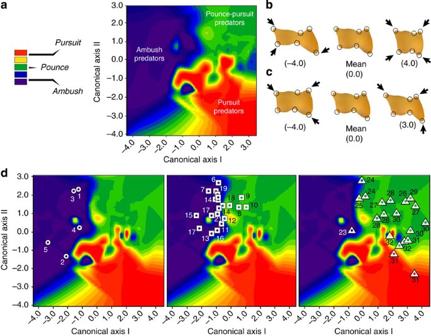Figure 2: Canonical variates analysis. (a) Contour plot depicted from the functions obtained in CVA performed from the elbow shape of living predators and the predatory grouping. (b) Elbow shape variation accounted for by the first canonical function. (c) Elbow shape variation accounted for by the second canonical function. Black arrows denote shape changes. (d) Contour plot depicted from the functions obtained in CVA performed from the elbow shape of living predators and the predatory grouping, but now including fossil forms. Number indicates species: 1,Hesperocyon gregarius; 2, Osbornodon fricki; 3, Mesocyon temnodon; 4, Enhydrocyon crassidens; 5, Mesocyon coryphaeus; 6, Archeocyon leptodus; 7, Archeocyon falkenbachi; 8, Phlaocyon leucososteus; 9, Cormocyonhaydeni; 10, Desmocyon thomsoni; 11, Cynarctus crucidens; 12, Psalidocyon marianae; 13, Epicyon saevus; 14, Epicyon haydeni; 15, Borophagus pugantor; 16, Borophagus parvus; 17, Borophagus secundus; 18, Carpocyon webbi; 19, Aelurodon asthenostylus; 20, Aelurodon mcgrewi; 21, Aelurodon taxoides; 22, Aelurodon ferox; 23, Leptocyon vulpinus; 24, Leptocyon vafer; 25, Leptocyon matthewi; 26, Vulpes stenognathus; 27, Urocyon minicephalus; 28, Eucyon davisi; 29, Canis thooides; 30, Canis armbrusteri; 31, Canis dirus; 32, Canis lupus. As indicated by the permutation test, both axes allowed a significant separation between the three pairs of predatory groups using both, the pairwise Mahalanobis distances and the pairwise Procrustes distances among groups ( Table 2 ; see also Supplementary Table 1 ). The first function ( Fig. 2a ) clearly distinguishes ambush predators from predators more specialized for running (that is, pounce-pursuit and pursuit, both known as cursorial) according to one set of morphological traits ( Fig. 2b ). The second function, however, separates both specialized predatory groups: pounce-pursuit predators from pursuit ones ( Fig. 2a ), showing a distinction between these two specialized hunting techniques according to a set of morphological traits ( Fig. 2c ). 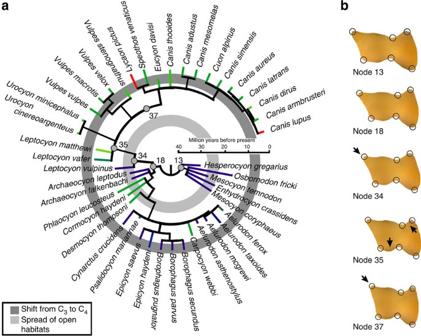Figure 3: Reconstruction of elbow-shape ancestral states. (a) Phylogeny of canids showing their temporal ranges (colours are the average scores obtained in CVA for each species. (b) Representation of ancestral elbow shapes using squared-changed parsimony26. Nodes 13, 18, 34 are the basal nodes for the three subfamilies, Node 35 is the basal for the tribe Canini plus Vulpini and, Node 37 is the basal for the tribe Canini typical of cursorial predators. Black arrows indicate morphological changes. The calculation of the scores for extinct canids ( Table 3 ) on both canonical functions provided a classification of fossil species into one of the three predatory groups according to their proximity to group centroids of extant carnivoran hunting techniques ( Supplementary Table 2 ). The inferred scores for the three subfamilies are plotted in Fig. 2d . Table 1 Sample size of extant carnivorans used in this study. Full size table Table 2 Results of the canonical variates analysis. Full size table Figure 2: Canonical variates analysis. ( a ) Contour plot depicted from the functions obtained in CVA performed from the elbow shape of living predators and the predatory grouping. ( b ) Elbow shape variation accounted for by the first canonical function. ( c ) Elbow shape variation accounted for by the second canonical function. Black arrows denote shape changes. ( d ) Contour plot depicted from the functions obtained in CVA performed from the elbow shape of living predators and the predatory grouping, but now including fossil forms. Number indicates species: 1, Hesperocyon gregarius; 2, Osbornodon fricki; 3, Mesocyon temnodon; 4, Enhydrocyon crassidens; 5, Mesocyon coryphaeus; 6, Archeocyon leptodus; 7, Archeocyon falkenbachi; 8, Phlaocyon leucososteus; 9, Cormocyon haydeni ; 10, Desmocyon thomsoni; 11, Cynarctus crucidens; 12, Psalidocyon marianae; 13, Epicyon saevus; 14, Epicyon haydeni; 15, Borophagus pugantor; 16, Borophagus parvus; 17, Borophagus secundus; 18, Carpocyon webbi; 19, Aelurodon asthenostylus; 20, Aelurodon mcgrewi; 21, Aelurodon taxoides; 22, Aelurodon ferox; 23, Leptocyon vulpinus; 24, Leptocyon vafer; 25, Leptocyon matthewi; 26, Vulpes stenognathus; 27, Urocyon minicephalus; 28, Eucyon davisi; 29, Canis thooides; 30, Canis armbrusteri; 31, Canis dirus; 32, Canis lupus. Full size image Table 3 Fossil data, museum numbers, geographical localities, and the subfamilies to which specimens belong as well as their stratigraphic ranges were taken from ref. 17 for the Hesperocyoninae, from ref. 18 for the Borophaginae and from ref. 19 for the Caninae. Full size table Furthermore, the result of the phylogenetic MANOVA of both canonical axes is significant for predatory behavior (Wilks=0.19018, F=15.517; P phyl =0.01598), which indicates that the difference between predatory groups in CVA is significant even after accounting for phylogenetic relationships. Elbow-shape ancestral states The reconstructed elbow shapes for the ancestors of the three subfamilies using the weighted squared-change parsimony algorithm [26] clearly resemble the unspecialized elbows of modern ambush predators ( Fig. 3 ; nodes 13, 18). However, while the basal hesperocyonines never evolved towards a more cursorial mode of hunting behaviour, the elbow morphologies of some derived borophagines were intermediate between those of living ambushers and the living pounce-pursuit canines, indicating some loss of supination in these forms ( Figs 2d , 3 ). Thus we conclude that the pounce-pursuit hunting technique evolved at least twice, independently within the Borophaginae and Caninae ( Fig. 3 ). In contrast, the reconstructed elbow shape for the ancestral node of the subfamily Caninae excluding the most basal canine sampled ( Leptocyon vulpinus ), that is, the ancestral state for the tribes Canini plus Vulpini (see Fig. 3 ), represents a step forward in locomotor specialization towards pounce-pursuit from the more basal borophagines to living canines ( Fig. 3 ; Node 35). Furthermore, a clear shift in elbow-joint shape occurred at the ancestral node of the tribe Canini ( Fig. 3 ; Node 37), representing the first appearance of elbow morphologies characteristic of fast-running canids over long distances. Figure 3: Reconstruction of elbow-shape ancestral states. ( a ) Phylogeny of canids showing their temporal ranges (colours are the average scores obtained in CVA for each species. ( b ) Representation of ancestral elbow shapes using squared-changed parsimony [26] . Nodes 13, 18, 34 are the basal nodes for the three subfamilies, Node 35 is the basal for the tribe Canini plus Vulpini and, Node 37 is the basal for the tribe Canini typical of cursorial predators. Black arrows indicate morphological changes. Full size image Body mass estimation The body masses of extant species ( Supplementary Table 3 ) regressed on the log-transformed centroid size resulted in highly significant line of best fit ( r =0.976; F=524.412; P <0.00001). The %PE was 18.28% and the % SEE was 25.75%. 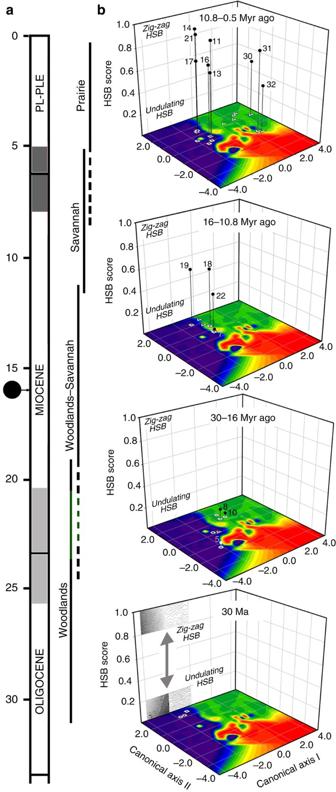Figure 4: Elbow-joint shape evolution in canids related to environmental change. (a) Major vegetational transitions trough the Cenozoic of North America11and major environmental events12,24. The light-grey box indicates the proposed timing for the spread of open-habitat grasses (23–27 Myr ago)12and the dark-grey box represent the shift in plant communities from C3 to C4 grasses (5–8 Myr ago)24. The black dot represent the Middle Miocene Climatic Optimum (MMCO) at 16 Myr ago35. (b) Three-dimensional morphospaces at different time intervals showing the relationship of elbow shape and the enamel layer arrangement (HSB) in extinct canids, as proxy for habitat openness. Each graph represents the mean of enamel data of those taxa present in different time intervals superimposed to their corresponding position inFig. 2c. Numbers denotes species:5, Mesocyon coryphaeus; 8, Phlaocyon leucososteus; 10, Desmocyon thomsoni; 11, Cynarctus crucidens; 13, Epicyon saevus; 14, Epicyon haydeni; 16, Borophagus parvus; 17, Borophagus secundus; 18, Carpocyon webbi; 19, Aelurodon asthenostylus; 21, Aelurodon taxoides; 22, Aelurodon ferox; 30, Canis armbrusteri; 31, Canis dirus; 32, Canis lupus. The predicted body mass values for extinct canids using the function generated from extant data are shown in Supplementary Table 4 . Although, the first species that reached or exceeded the postulated threshold value in carnivore biology of 21.5 kg for which species are able to take prey as large as, or larger than, themselves was the hesperocyonine Osbornodon fricki at ∼ 15–18 Myr ago, species exceeding this physiological threshold were not common until the appearance of the Aelurodontina and Borophagina subtribes of the subfamily Borophaginae at ∼ 15–7 Myr ago. Finally, within the subfamily Caninae, species reaching or exceeding the 21.5 kg threshold were common at the beginning of the Pleistocene with the appearance of some species of the genus Canis at around 2 Myr ago. Enamel specialization The results of the analysis on the enamel Hunter–Schreger band (HSB) specialization in canids are shown in Supplementary Table 5 . In summary, hesperocyonine canids exhibit little or no development of acute or zig-zag angles in their cheek dentitions. In contrast, the initial increase in degree of HSB specialization occurred around ∼ 23–22 Myr ago in borophagine canids and in the large and specialized Enhydrocyon crassidens . By ∼ 15 Myr ago, HSB scores of >0.4 were common among borophagines, and fully zig-zag enamel prism bands (with the maximum HSB score of 1) appeared around 12–10 Myr ago in borophagines such as Aelurodon taxoides . The broad range of HSB scores represented by borophagine species and late Miocene canine species are maintained by Pleistocene and extant canines after the extinction of borophagines by the end of the Pliocene. Both of the canonical axes distinguished the extant forms into the three predatory behavioural groups ( Fig. 2a ; Supplementary Table 1 ). Furthermore, changes in elbow-joint shape captured by each axis show the morphological adaptations for different types of predatory behaviour: ambush predators retain the generalized mammalian condition of relatively wide joints with high supinatory abilities, enabling grappling with the prey; pursuit predators have narrow and ‘box-like’ elbows with limbs locked into a more prone position; and the elbow-joint morphology of pounce-pursuit predators is somewhat intermediate, but with some unique features [22] ( Fig. 2b,c ). It should be noted that, to a certain extent, among cursorial predators, pounce-pursuit versus pursuit behaviour is related to body size (but see ref. 22 ): smaller carnivores (>20 kg) are pounce-pursuit predators and larger ones are pursuers, but some large pounce-pursuit predators exist (for example, dingoes and the striped and brown hyenas). When both of the canonical functions are applied to fossil taxa they indicate a directional change in elbow-joint shape over the past ∼ 37 Myr ago: from that reflective of wide joints among the basal hesperocyonines, through the intermediate-shaped joints of borophagines, to the more ‘box-like’ elbows of the Recent more derived canines ( Fig. 2d ), reflecting increasingly restricted forearm rotation. However, as evidenced by the reconstructed elbow shapes for the ancestors of the three canid subfamilies using parsimony-based algorithms, the basal hunting mode in all three canid clades was the more generalized ambush condition ( Fig. 3a,b ). A qualitative proxy for cursorial abilities in living and extinct canids that supports our CVA results is the degree of reduction of the entepicondylar foramen in the anterior distal epiphysis of the humerus ( Fig. 1a ) as the degree of foramen reduction parallels other changes in forelimb morphology for cursorial efficiency [27] . In fact, although all hesperocyonines have a well-developed foramen and borophagines plus the primitive canine Leptocyon vulpinus have an intermediately developed foramen, other more specialized cursorial canines greatly reduce the foramen ( Supplementary Fig. 2 ). This progressive reduction through the evolution of canids seems to be associated with a progressive restriction in forearm supination—a direct consequence of acquiring cursorial specialization. However, the absence of this entepicondylar foramen in some highly derived species of the genus Borophagus (see Supplementary Fig. 2 ) supports the evidence that the ambush type of predation secondarily evolved in large and derived borophagine canids. Tracing changes of elbow-joint shape through time indicates that until ∼ 30 Myr ago only ambush canids were present ( Fig. 4b , 30 Myr ago). Given that closed habitats today harbour mainly ambush predators [23] , this morphology accords with the predominant Oligocene habitats dominated by woodlands [12] . This is also evidenced by the analysis of canid enamel microstructure, as these taxa did not experience any increasing of HSB folding in their teeth ( Fig. 4b , 30 Myr ago), indicating that early borophagine or hesperocyonine canids were not adapted to feed on bone (from carcasses) or inadvertently ingesting significant amounts of grit [28] , both being items that are facilitated by the expansion of open environments [29] , [30] , [31] , [32] . Figure 4: Elbow-joint shape evolution in canids related to environmental change. ( a ) Major vegetational transitions trough the Cenozoic of North America [11] and major environmental events [12] , [24] . The light-grey box indicates the proposed timing for the spread of open-habitat grasses (23–27 Myr ago) [12] and the dark-grey box represent the shift in plant communities from C3 to C4 grasses (5–8 Myr ago) [24] . The black dot represent the Middle Miocene Climatic Optimum (MMCO) at 16 Myr ago [35] . ( b ) Three-dimensional morphospaces at different time intervals showing the relationship of elbow shape and the enamel layer arrangement (HSB) in extinct canids, as proxy for habitat openness. Each graph represents the mean of enamel data of those taxa present in different time intervals superimposed to their corresponding position in Fig. 2c . Numbers denotes species: 5, Mesocyon coryphaeus; 8, Phlaocyon leucososteus; 10, Desmocyon thomsoni; 11, Cynarctus crucidens; 13, Epicyon saevus; 14, Epicyon haydeni; 16, Borophagus parvus; 17, Borophagus secundus; 18, Carpocyon webbi; 19, Aelurodon asthenostylus; 21, Aelurodon taxoides; 22, Aelurodon ferox; 30, Canis armbrusteri; 31, Canis dirus; 32, Canis lupus . Full size image In fact, palaeosols and fossil phytolith assemblages indicate that open habitats dominated by grasses were not common in North America until the latest Oligocene [12] . Our results indicate that this time was coincident with the first appearance of pounce-pursuit canids also adapted to an abrassive diet based on the combined elbow shape and enamel microstructure data. The earliest species classified by the CVA as incipient pounce predators were the small borophagines Cormocyon haydeni (ca. 3.6 kg; ∼ 19–29 Myr ago), Desmocyon thompsoni (ca. 10.5 kg; ∼ 17.5–24 Myr ago) and Phlaocyon leucosteus (ca. 3.7 kg; ∼ 16–22 Myr ago), coincident with proposed timing for the spread of grasses ( Figs 2d , 3 ; Supplementary Table 2 ). Studies of carbon isotope composition of palaeosols attest that this initial spread of grasses was due to the expansion of C 3 grasses over trees and shrubs, resulting in C 3 dominated ecosystems [33] , [34] . Some of these taxa show an initial increase of HSB folding ( Fig. 4b , 30–16 Myr ago), which indicates some consumption of abrasive and/or hard items (grit or bone) typical of more open habitats [28] , [29] , [30] , [31] , [32] by these late Oligocene-early Miocene taxa. The increasing HSB folding in the teeth of the derived hersperocyonine Enhydrocyon crassidens (ca. 18.3 kg; ∼ 19–29 Myr ago) indicates that this ambush predator also inhabited in woodlands–savannahs ( Fig. 4b , 30–16 Myr ago) as living lions do today. Therefore, our data suggest that canids with specialized hunting techniques and durophagous diets of more open environments first appeared in accord with the proposed timing for the spread of grasses indicated by phytolith data [12] . From the Middle Miocene Climatic Optimum [35] ( ∼ 16 Myr ago; MMCO; Fig. 4a ) to the Late Miocene ( ∼ 10.8 Myr ago) the diversity of pounce-pursuit canids increased, mainly due to the diversification of the subfamily Caninae. Following the MMCO, open habitats also increased in association with declining temperatures and increasing aridity [10] , [35] –an environmental pattern also tracked by the significant increase in the HSB folding of teeth enamel in post-MMCO taxa ( Fig. 4b , 16–10.8 Myr ago). During the Late Miocene and Early Pliocene, this climatic and environmental trend was accompanied by an increasing specialization towards more cursorial abilities and more durophagous habits in canids, indicating that these taxa inhabited more open environments. In fact, the first appearance of elbow morphologies indicative of a pounce-pursuit behaviour and a high degree of HSB folding within canines took place at this time ( Figs 2d , 3 and 4b , 10.8–0.5 Myr ago). The pounce-pursuit behaviour first appeared in canine canids with some small-sized forms such as Leptocyon matthewi ( ∼ 12.6–9 Myr ago) or Leptocyon vafer ( ∼ 14–9 Myr ago; Fig. 4 ; Supplementary Table 4 ) and the reconstructed elbow shape for the ancestral state of the tribes Canini plus Vulpini within the subfamily Caninae indicates a clear shift in elbow morphology towards the behavior of pounce-pursuit predators (Node 35; Fig. 3 ). However, elbow morphologies typical of modern pounce-pursuit predators first appear with early precursors of modern foxes (that is, Vulpes stenognathus ) and an ancestral genus of modern canines (that is, Eucyon davisi ) at ∼ 5–9 Myr ago [36] , as these taxa are the first that occupy a central position (not a peripheral position) in the morphospace of modern pounce-pursuit predators ( Fig. 4b , 10.8–0.5 Myr ago). Therefore, our data suggest an association between environmental change and predatory behaviour, as this time was coincident with a marked shift in the dominant photosynthetic pathway of grasses [24] —from C 3 to C 4 —in turn associated with the spread of extremely open savannas or prairies ( Fig. 4a ). The carbon isotope composition of palaeosols confirms that C 4 grasses were not expanded until the late Miocene or early Pliocene in North America [33] , [34] . However, the large canids of the late Miocene, borophagines such as Epicyon or Borophagus , do not show any trend towards the morphology of a pursuit, as most probably, they secondarily reverted to more ambush-like elbow morphology, reflecting greater specialization at a larger body sizes ( Fig. 3 ). The coexistence of these large ambush borophagines with the earliest pounce canines suggests a diversity of habitats in North America at this time. In fact, palaeosol data indicate habitats composed by C 3 trees and shrubs over a carpet a C 4 grasses [33] , [34] . Finally, following the extinction of the subfamily Borophaginae, during the Pleistocene, members of the subfamily Caninae evolved large body sizes, echoing the trend seen in both of the extinct subfamilies to become larger and more carnivorous over time [36] , [37] . This evolutionary size increase, initially seen in the specialized late Miocene pounce-pursuit members of the Caninae, led to the emergence during the Pleistocene of large sized ( ∼ 50 kg; Fig. 4c ; Supplementary Table 4 ) long-distance pursuit predators, with the appearance in North America of the grey wolf Canis lupus and the extinct dire wolf Canis dirus ( Figs 2d , 3 and 4b , 10.8–0.5 Myr ago). This result was confirmed by the reconstruction of the ancestral state of the tribe Canini whose shape clearly resembles the elbows of long-distance pursuit predators ( Fig. 3b ). The appearance of pursuit predatory behaviour was also coincident with the appearance of a degree of HSB folding in canine canids comparable to the HSB folding of earlier borophagines ( Fig. 4b , 10.8–0.5 Myr ago). This suggests that the later specialized pursuit predators were adapted to inhabit extremely open prairies dominated by C 4 grasses [33] , [34] . As indicated by carbon isotope composition of palaeosols, this time was coincident with levels of C 4 grasses biomass (>50%) like those in some regions of North America today (that is, Great Plains) [33] , [34] . In fact, around the same time other possible pursuit predators [13] , such as the cheetah-like felid Miracinonyx or the fast-running hyena Chasmaporthetes , immigrated to North America from Eurasia [16] . Our results indicate that mammalian herbivores were not the only groups strongly influenced by Cenozoic climatic change and its impact on vegetation and habitat structure. Predators change their predatory habits when herbivores change their foraging behaviour in association with habitat opening related to climatic change. The marked response to environmental transformation by late Cenozoic canids reported here demonstrate that long periods of profound climatic change are critical for the emergence of ecological innovations and could alter the direction of lineage evolution. Materials, landmarks and geometric morphometrics The elbow-joint shape in the 139 specimens (92 living specimens distributed among the families Felidae, Hyaenidae, Viverridae, Mustelidae and Canidae of the order Carnivora ( Table 1 ) and 47 fossil specimens of the family Canidae including representatives of the three subfamilies, Hesperocyoninae†, Borophaginae† and Caninae [17] , [18] , [19] ( Table 3 ) was recovered by digitizing six landmarks in 2D on the anterior surface of the humerus distal epiphysis [20] , [21] , [22] from high-resolution digital images ( Fig. 1a ). The digital images were taken with a tripod and following a standardized protocol for avoiding lens distortion and parallax. We sampled those families of living carnivores with large representatives such as canids, felids and hyenids, because the inclusion of viverrids and mustelids do not add crucial information in terms of body size or predatory behaviour. However, we also sampled the wolverine because it is the largest mustelid ( Gulo gulo ), an ambush predator, and the large African ( Civettictis civetta ) and Indian ( Viverra zibetha ) civets. The six landmarks were digitized into 2D Cartesian coordinates ( x , y ) using TPSdig V. 211 (ref. 38 ; Supplementary Data 1 ) but we modelled the inter-landmark distances by means of an outline to obtain clearer shape transformation models in subsequent multivariate analysis. In addition, we superimposed the 2D outlines into a three-dimensional scanned surface of a jaguar, Panthera onca (139959, AMNH) specimen to obtain clear interpretations of the shape transformation recovered in the axes derived from different multivariate approaches. All the specimens digitized were aligned using Procrustes and projected onto the tangent space [39] . The size of the specimens was represented by their centroid size (Cs), which allows post-hoc assessment for allometric effects [40] . Centroid size is the square root of the sum of squared distances of each landmark from the centroid of the configuration [40] . The calculation of Procrustes Coordinates (Proc) and Cs were performed with MorphoJ [41] . We used the same six landmarks as Andersson [20] , as they are established morphological indicators of forearm pronation and supination. However, whereas Andersson [20] analysed solely the Euclidean distances among landmarks, we used an approach based on Geometric Morphometrics. Our approach not only captures the relative distances among the landmarks, but also the topological information contained within them. The influence of size and phylogeny in elbow-joint shape We assembled a phylogenetic consensus tree ( Supplementary Fig. 1 ) following various published sources using Mesquite [42] . We incorporated branch lengths in our composite phylogeny in million years before present [43] , [44] . In the case of living species, branches were scaled according to node dates estimates based on Nyakatura and Bininda–Emonds [45] . In the case of extinct taxa, fossil occurrence dates were compiled from various sources based on species locality and age information ( Table 2 ), and the branch lengths were estimated from the first and last appearance of taxa ( Supplementary Fig. 1 ). We used this phylogenetic tree to assess phylogenetic patterning in our data. As we are only interested in quantifying the presence of phylogenetic signal, instead of the strength of the phylogenetic signal, we used the permutation approach developed by Laurin [46] , extended for multivariate analysis by Klingenberg and Gidaszewski [47] , and applied to shape data by other authors (for example, refs 48 , 49 , 50 , 51 , 52 , 53 , 54 ), to simulate the null hypothesis of complete absence of phylogenetic signal in elbow shape. The mean species shapes are randomly distributed as the tips of the phylogeny in 10,000 permutations, and for each permutation, the tree length was computed. If the resulting tree length computed for each permutation was greater than the one obtained with the original data, the null hypothesis of absence of phylogenetic structure was rejected. A P -value was used for assessing the presence of phylogenetic signal in shape [47] . A multivariate regression analysis [55] of shape (that is, using Proc) on size (that is, using Cs) was performed to test the influence of allometry. In addition, we applied independent contrasts analysis [56] to take into account the phylogenetic relationships of the species under study. Following this, we regressed the contrast for shape (Proc) on the contrast for size (Cs) using MorphoJ [41] . The statistical significance of both multivariate regression analyses was tested with a permutation test against the null hypothesis of complete independence of shape on size [57] . We performed a multivariate regression analysis [55] of the independent contrast of the Proc against the s.d. of the standardized contrast (that is, the square root of the corrected branch lengths) with MorphoJ [41] , following Díaz-Uriarte and Garland [25] . The values of the s.d. were obtained from the PDAP module for Mesquite [42] , [58] . The significance of this regression was evaluated with a permutation test against the null hypothesis of complete independence between the two variables. This test was specifically performed to explore the adequacy of: (i) the model used for tree topology; (ii) the branch lengths used; and (iii) the model of Brownian motion for our tip data [25] . Inferring predatory behaviour in extinct canids To determine those elbow-joint shape features that best distinguish among the three present-day predatory modes (ambush; pounce-pursuit; and pursuit), we performed a CVA from the Proc of elbow shape in modern predators. We used CVA instead of Principal Components Analysis (PCA) as performed by Andersson [20] because to find those elbow-shape features that best distinguish among these predatory groups of specimens, the use of CVA is more appropriate than PCA. In fact, while CVA is a classification method, PCA is an ordination one. In any case, it is worth mentioning that although Andersson [21] also used CVA, the analysis was performed to differentiate among the three subfamilies of canids instead to infer their predatory behaviour. We classified all of the living species into one of the three present-day predation modes following previously published sources [23] , [59] as follows: (i) ambush predators stalk their prey and may pursue them over short distances, and the forelimbs may be used to grapple with large prey; (ii) pounce/pursuit predators usually hunt small prey using either a pounce or short chase, and rarely grapple with their prey; And (iii) pursuit predators usually chase their prey for a long distance (>30 m), and may hunt cooperatively to bring down large prey, but do not grapple with their prey ( Table 1 ). Therefore, we consider here the pounce-pursuit category of Van Valkenburgh [23] instead of only ‘cursorial’ and ‘non-cursorial’ predators as Andersson [20] differenced. However, these three hunting types are usually correlated with prey size, while ambushers can take prey of all sizes, pounce predators usually take small prey and pursuit predators usually take large prey. Both ambush and pursuit predation can be directly linked to forearm mobility and elbow function in the case of large prey, but a predator will not ‘pounce’ on large prey nor ‘pursue’ small prey. We consider the cheetah ( Acinonyx jubatus ), the only highly cursorial felid, to be a pursuit predator, even though this species still retains some ability to supinate as they often swat their prey (but they do not grasp it). The reason is because the cheetah is a solitary hunter but does not have the endurance of the canid and hyenid pursuit predators and it will bring down its prey with the swipe of a forelimb. However, the cheetah is a felid that is clearly more specialized towards running than others in its family, pursuing its prey for a distance of up to 200 m and it has been classified as a pursuit predator by other researchers [15] , [59] . As the predatory categories used here are dynamic and not static, our predatory grouping scheme established by Van Valkenburgh [23] represents an arbitrary division of a continuous range. Furthermore, many carnivorous taxa range over some predatory types (for example, the cheetah), and so the assignment of a given species to a particular category is a ‘best fit’ designation rather than an exclusive one. In summary, our predatory categories are thus a significant (albeit necessary) simplification of the complex range of predatory behaviour. The reliability of group separation was assessed by the pairwise Procrustes distances and Mahalanobis distances among all possible pairs of groups using the pooled within-group covariance matrix for all the groups jointly. A permutation test was computed for the Mahalanobis and Procrustes distances of all pairwise comparisons. The statistical significance of these pairwise differences was assessed with 10,000 permutations using MorphoJ [41] . Both canonical functions obtained from the living sample in CVA were later applied to fossil taxa using their Proc of elbow shape. However, although we will never be sure if the established predatory categories based on living carnivores can be extrapolated to extinct species, this uncertainty is alleviated if fossil forms have extant relatives. This is particularly the case of the family Canidae, as extant forms phylogenetically bracket them, where the morphological correlates of behaviour are known. We used the direct method of leave-one-out cross-validation for assessing the percentage of probability of living canids to belong for one of the three present-day predation modes. The classification of fossil species into one of the three predatory groups was inferred according to their proximity to group centroids of the three predatory groups of extant carnivorans with SPSS v.19. We did not use the stepwise discriminant analysis [60] because we have more cases per group than predictor variables; 12 variables or six bi-dimensional landmarks digitized in 35 pounce-pursuit predators, 30 ambush predators and 22 pursuit predators ( Table 1 ). Thus, there is no statistical reason to perform a stepwise approach instead of the direct method because CVA only tends to over fit differences in those cases where there are more variables than the number of cases within groups [61] . The morphospace depicted from the scores of the living specimens into both canonical axes was imported into the graphing software SigmaPlot to create a contour plot that was colour coded by predatory mode—extant ambushers in blue, extant pounce-pursuit predators in green and extant pursuit predators in red. Colour degradation within each predatory group was calibrated to the frequency of the specimens within each predatory group. After we performed this contour plot from the scores of the living taxa, we repeated the same graphs but now including the fossils according to their predicted predatory category obtained in CVA. We recovered a RGB colour code for each fossil specimen according to its position in the contour plot living morphospace. To test whether carnivores with different predatory behaviour differed in shape irrespective of phylogeny, we used the aov.phylo function in the R package ‘geiger’ [62] using both canonical axes. We used Brownian motion as a model for evolutionary change and ran 1,000 simulations to create an empirical null distribution to compare with our sample. Ancestral elbow-shape reconstruction All taxa excluding canids were pruned from the phylogenetic tree shown in Supplementary Fig. S1 using Mesquite [42] . The ancestral states, or internal phylogenetic nodes, were reconstructed by squared-change parsimony [26] weighted by branch lengths using MorphoJ [41] . The main purpose to reconstruct ancestral states was to explore patterns of elbow-joint shape evolution and by extension the evolution of predatory behaviour in canids. Also, we would be able to assess the most probable basal hunting technique for the three subfamilies and when the specialized traits of the elbow are acquired through the evolution of canids. Body mass estimation in extinct taxa To explore if elbow-shape changes experienced by the evolution of the family could be in part explained by a previously reported trend towards size increase through canid evolution [37] , we explored the issue of whether the appearance of canids with morphology indicative of more cursorial behaviour (pounce-pursuit or pursuit) is the result of their body mass reaching or exceeding 21.5 kg, which is a threshold value in carnivore biology: only carnivores of this size or greater take prey as large as, or larger than, themselves [63] . We estimated the body masses (BMs) of fossil canids by means of a least-square bivariate regression of log-transformed BM on Cs for the extant taxa (log (BM)=a+bLog[Cs]) using SPSS v.19. Although both body mass and elbow centroid size are variables, each with its own errors and distributions under the control of the investigator, we chose the least-square regression model (instead of a type II) because our purpose here was to explore the body mass dependency of elbow centroid size. Note that the main objective here was to obtain a model in which body mass can be predicted from elbow centroid size. For these reasons, we assumed dependence between both variables [64] . The body mass for each extant species was taken from recent studies on body mass estimation in extinct taxa [64] , [66] and references therein. Their Cs were then computed as the Cs average for all the specimens belonging to the same species. The accuracy of the bivariate regression function was evaluated by means of the F -statistic and Pearson’s correlation coefficient ( r ). However, as the correlation coefficient can be high even with high residuals [67] , it is not a highly appropriate statistic to evaluate the predictive power of a regression equation. Thus, to evaluate the predictive power of the function, we computed the per cent prediction error (%PE) and the per cent standard error of the estimate (%SEE) [67] . Once we had confirmed the significance of the Log-BM on Log-Cs regression equation and its predictive power, we predicted body mass values for the extinct canids. Enamel microstructure specialization in extinct canids The association between environmental change and canid predatory behaviour was investigated using the arrangement of the enamel prism bands—known as bands of Hunter–Schreger (HSB)—as a proxy. The reason is because carnivores that live in open environments consume more intrinsic (bones from carcasses) and extrinsic (grit) hard food items, which relates to heavily folded HSB [28] , [51] , [68] , [69] , [70] . Studies of carnivorans demonstrate a link between bone and carcass consumption and increased kleptoparasitism in open habitats because of increased carcass detectability [30] , [31] , [32] . Therefore, we utilize HSB analysis as proxy of habitat openness, in terms of increased enamel resistance to wear from ingested grit, as well as hard vertebrate tissue consumption associated with increased carcass availability in open environments. To quantify the degree of specialization in the enamel prism bands arrangement (bands of Hunter–Schreger; HSB), we used a stereomicroscope at 5–40 × magnification. We coded for each tooth in the dentition, the degree of HSB specialization in each of the three regions on the tooth crown (base, tip, and the mid region), each occupying approximately one-third of total crown height. We quantified the degree of HSB specialization as follows: the less-specialized undulating pattern; then the intermediate acute-angled undulating pattern; and followed by the most specialized zig-zag HSB pattern [70] . The final data set included both newly collected data as well as published data in Tseng [69] ( Supplementary Table 5 ). The coded HSB pattern for each tooth was given as a score from 0 (for undulating pattern in all three regions of the tooth crown) to 1 (for zig-zag pattern in all three regions of the crown). We studied lower cheek dentitions (premolars and molars) of fossil canid species. However, we used the upper dentitions for those species without preserved dentaries. Furthermore, where both left and right dentitions were available, averages of scores were taken across the corresponding tooth and treated as a single entry in the data analysis. Because not all fossil specimens contained complete data for the premolar–molar sequence, 10% of the data set represent composite HSB data from multiple specimens of the same species. The final HSB score for each specimen data point was calculated per tooth (total HSB score divided by number of teeth coded per specimen) to account for differences in completeness and tooth count of sampled species ( Supplementary Table 5 ). How to cite this article: Figueirido, B. et al. Habitat changes and changing predatory habits in North American fossil canids. Nat. Commun. 6:7976 doi: 10.1038/ncomms8976 (2015).